Structural basis for the recognition and cleavage of histone H3 by cathepsin L Proteolysis of eukaryotic histone tails has emerged as an important factor in the modulation of cell-cycle progression and cellular differentiation. The recruitment of lysosomal cathepsin L to the nucleus where it mediates proteolysis of the mouse histone H3 tail has been described recently. Here, we report the three-dimensional crystal structures of a mature, inactive mutant of human cathepsin L alone and in complex with a peptide derived from histone H3. Canonical substrate–cathepsin L interactions are observed in the complex between the protease and the histone H3 peptide. Systematic analysis of the impact of posttranslational modifications at histone H3 on substrate selectivity suggests cathepsin L to be highly accommodating of all modified peptides. This is the first report of cathepsin L–histone H3 interaction and the first structural description of cathepsin L in complex with a substrate. Cathepsin L is one of 11 human cysteine cathepsin proteases, which share a catalytic mechanism and strong sequence similarity with the non-specific plant protease, papain [1] . All members of this cathepsin family contain lysosomal targeting motifs, exhibit maximal activity at acidic pH and utilize autocatalytic activation mechanisms. Cathepsin L predominantly exhibits endoprotease activity that is essential for limited endosomal and lysosomal proteolysis, making it an important contributor to both protein degradation [1] and development and function of the immune system [2] , [3] . Despite their predominant lysosomal localization, a role for these proteases, including cathepsin L, in the nucleus has been reported. For example, the nuclear serpin myeloid and erythroid nuclear termination stage-specific protein is a potent chromatin remodelling protein that also efficiently inhibits cathepsins V and L [4] , [5] , [6] , [7] , [8] . Stefin B (cystatin B), another endogenous inhibitor of cysteine proteases, specifically interacts with histones H2A.Z, H2B, H3 and cathepsin L in the nuclei of T98G astrocytoma cells [9] . A serpin A3G, upon classical but not alternative activation of macrophages, exhibits increased localization in the nucleolus and colocalization with cathepsin L [10] . Nuclear variants of cathepsins B and V are involved in the development of thyroid malignancies by modifying DNA-associated proteins [11] . A role for cathepsin L in cleavage of the CUX1 transcription factor and the resultant acceleration of cell-cycle progression into S phase has also been described [12] , [13] , [14] . Furthermore, cathepsin L deficiency is correlated with a global rearrangement of chromatin structure and a redistribution of posttranslationally modified histones [15] . Though the specific mechanisms underlying the nuclear localization remain unclear, translocation has been associated with both truncated and proteolytically processed forms of the protease [12] , [16] . In addition to targeting transcription factors, nuclear proteases have been shown to target the tail of histone H3 in yeast and mice [16] , [17] . In both organisms, A21 from the H3 tail appears to be the primary site for proteolytic processing. Though the yeast endopeptidase has yet to be identified, the nuclear activity from mice has been attributed to the cysteine protease, cathepsin L [16] . Crystallographic work has so far been centred on inhibitor-bound complexes of the mature, active enzyme as well as on the structures of inactive cathepsin mutants with intact prosegments [18] , [19] , [20] , [21] , [22] . In this work, we have utilized a mature form of cathepsin L with the active site residue C25 mutated to alanine (referred to as mC25A hereafter) for our structural studies. We report the first structural characterization of a cathepsin family member in complex with a cognate substrate, a peptide derived from the human histone H3 tail ( Supplementary Fig. S1 ). Furthermore, we have explored the effects of peptide length, mutations and posttranslational modifications (PTMs) of histone H3 on cleavage by cathepsin L. Cathepsin L active site is unperturbed by the C25A mutation The structure of the apo form of the mature C25A cathepsin L mutant, termed as apo-mC25A, was determined to 2.2 Å by molecular replacement using the wild-type structure of cathepsin L (derived from PDB 3BC3 ) [18] as a search model ( Fig. 1a ). Comparison of apo-mC25A with previously determined structures from the cathepsin family yielded excellent alignment with the mature forms of cathepsins K, L and S, for which the r.m.s. deviations range from 0.6 to 0.8 Å over >200 aligned residues ( Fig. 1b ). Close inspection of the active site cleft of apo-mC25A reveals little structural difference compared with the wild-type active form ( Fig. 1b ). 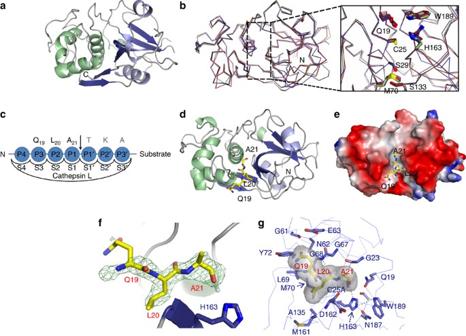Figure 1: Crystal structures of apo-mC25A and the mC25A and histone H319−33peptide complex. (a) The crystal structure of the apo form of the mature, inactive cathepsin L mutant, mC25A. (b) Alignment of the apo-C25A structure with other cathepsin structures of PDB codes1NPZ,1VSNand3BC3reveals no perturbation in global structure or on the conformation of residues comprising the active-site cleft on mutation of the catalytic cysteine. (c) The standard nomenclature designating the peptide-binding subsites of the cathepsin L active-site-binding cleft. The substrate residues apparent in the crystal structure are indicated in bold. (d) The crystal structure of the mC25A cathepsin L mutant in complex with a peptide derived from the human H3 tail corresponding to residues 19–33 of histone H3 (QLATKAARKSAPATG). Only residues Q19, L20 and A21 could be placed. (e) The Q19–A21 segment of the substrate peptide was fitted into unprimed subsites. The electrostatic surface of mC25A is shown with regions of negative charge indicated in red and positive charges in blue. (f) The Fo–Fc difference density at 3σ contour. The placement of L20 in the S2 subsite was unambiguous. (g) The H3L20 residue occupies the S2 subsite, where it makes a variety of van der Waals contacts with the indicated mC25A side chains. As predicted from biological data, H3A21 occupies the S1 subsite where the S1–S1′ peptide bond would be oriented for nucleophilic cleavage. Figure 1: Crystal structures of apo-mC25A and the mC25A and histone H3 19−33 peptide complex. ( a ) The crystal structure of the apo form of the mature, inactive cathepsin L mutant, mC25A. ( b ) Alignment of the apo-C25A structure with other cathepsin structures of PDB codes 1NPZ , 1VSN and 3BC3 reveals no perturbation in global structure or on the conformation of residues comprising the active-site cleft on mutation of the catalytic cysteine. ( c ) The standard nomenclature designating the peptide-binding subsites of the cathepsin L active-site-binding cleft. The substrate residues apparent in the crystal structure are indicated in bold. ( d ) The crystal structure of the mC25A cathepsin L mutant in complex with a peptide derived from the human H3 tail corresponding to residues 19–33 of histone H3 (QLATKAARKSAPATG). Only residues Q19, L20 and A21 could be placed. ( e ) The Q19–A21 segment of the substrate peptide was fitted into unprimed subsites. The electrostatic surface of mC25A is shown with regions of negative charge indicated in red and positive charges in blue. ( f ) The Fo–Fc difference density at 3σ contour. The placement of L20 in the S2 subsite was unambiguous. ( g ) The H3L20 residue occupies the S2 subsite, where it makes a variety of van der Waals contacts with the indicated mC25A side chains. As predicted from biological data, H3A21 occupies the S1 subsite where the S1–S1′ peptide bond would be oriented for nucleophilic cleavage. Full size image Crystal structure of the mC25A-H3 19−33 complex The papain-like cysteine proteases, including cathepsin L, possess substrate-binding pockets that can be divided into seven binding subsites, S4 to S3′, that interact with distinct amino acids of the target substrate and confer substrate specificity ( Fig. 1c ). The inactive mC25A cathepsin L mutant was cocrystallized with a histone H3 peptide covering residues 19–33 of the human histone H3 tail ( Fig. 1d,e ). Electron density was only apparent for residues Q19, L20 and A21, which occupy the unprimed region (subsites S3, S2 and S1, respectively) of the cleft ( Fig. 1f ). Electron-density difference map calculations revealed excellent electron densities corresponding to the backbone region of this peptide segment and to the side chains of L20 and A21 at a contour level of 3σ. Difference electron density for the Q19 side chain is apparent at the 2σ contour. Systematic shifting of the peptide register throughout the active-site cleft placing other amino acids in the S2 subsite produced less satisfactory results during modelling and refinement ( Supplementary Fig. S2 ). Thus, the apparent difference electron density coupled with the known preference for hydrophobic residues at the S2 subsite and other biochemical data reported in this study and elsewhere [16] led to the final modelling of the QLA peptide in the active-site cleft. No electron density was present to support the placement of peptide residues along the primed region of the active-site cleft, even at low sigma contours. The P1 residue, H3A21, is involved in a highly connected network of hydrogen bonds, which anchors its carbonyl oxygen atop the imidazole ring of H163, the general base in the catalytic reaction. The amide nitrogen of the H3A21 residue engages in hydrogen bonding with the carbonyl oxygen of mC25A-D162 ( Fig. 1g ). The carbonyl oxygen of H3A21 forms a hydrogen bond with the ND1 atom of the catalytic H163 ( Fig. 1g ). The conformation of H163 from cathepsin L is further restricted through its hydrogen bond interactions with N187 and W189. The β-carbon of the H3A21 residue points directly upward from the base of the active-site cleft and makes no specific interactions, thus permitting substitution at this site without significant impact on the substrate suitability ( Fig. 1e,g ). The side chain of the P2 residue, H3L20, makes a number of favourable van der Waals contacts with the residues lining the S2 subsite, including the side chain atoms of L69, M70 and A135, and the main chain atoms of H163 and D162 ( Fig. 1g ). This residue is additionally constrained through the formation of main chain hydrogen bonds with G68 of cathepsin L. In contrast to the narrow S2 subsite, which restricts the recognition of substrate residues, much more conformational plasticity is permissible for the S3 subsite. No specific interactions are recognizable between the P3 residue H3Q19 and cathepsin L, despite the presence of electron density supporting its ordered placement. General van der Waals contacts are made with residues lining the lower region of the cleft: G61, E63, L69 and Y72 ( Fig. 1g ). H3L20 recognition by cathepsin L is essential for activity The ability of human cathepsin L to cleave peptides derived from histone tails was assessed by both direct activity measurement using intramolecularly quenched fluorogenic (IQF) peptides ( Table 1 ) and competition assays using the commercial Z-LR-4-methyl-7-coumarylamide (Mca) substrate ( Tables 2 and 3 , Supplementary Tables S1 and S2 ). 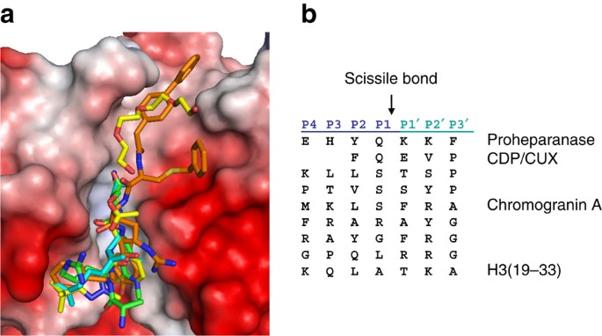Figure 2: Structural and sequence alignment of inhibitors and substrate sequences in the cathepsin L cleft. (a). Superimposition of the H319−33(cyan) peptide with the cathepsin L inhibitors, AZ12878478 (yellow, PDB3HHA), and S-benzyl-N-(biphenyl-4-ylacetyl)-L-cysteinyl-N′5′-(diaminomethyl)-D-ornithyl-N-(2-phenylethyl)-L-tyrosinamide (orange, PDB3BC3). In addition to the AZ12878478, an acetate ion aligning with the catalytic residues and a polyethylene moiety in the prime region were also modelled. (b) Sequence alignments of selected cathepsin L substrates as identified by mass spectrometry. Each protein target is subject to multiple site of cleavage with both canonical and atypical substrate recognition by the S2 pocket, though consistently there is preference for large and bulky hydrophobic side chains at the S2 site. The loss of competitive inhibition for the H3 14−31 L20A and H3 14−31 Q19A/L20A mutant peptides in our assays further underscores the importance of leucine recognition in substrate turnover ( Table 2 and Supplementary Table S1 ). Mutation of Q19 to alanine in H3 14−31 ( Supplementary Table S1 ), however, had no discernable effect on proteolytic processing activity, which also supports the placement of L20 in the S2 subsite of our mC25A-H3 19−33 complex structure. 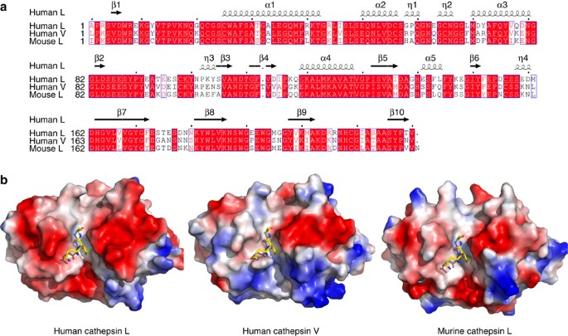Figure 3: Sequence and structural conservation among human cathepsins L and V and murine cathepsin L. (a) Structure-based sequence alignment of cathepsins L and V. White residues on red background indicate identical residues, red residues on white represent similar residues and the other residues are coloured in black. (b) Surface representation of human cathepsins L, V and murine cathepsin L. The structure of murine cathepsin L is modelled based on human cathepsin L. The histone H3 peptide in human cathepsin L complex structure is superimposed to human cathepsin V and murine cathepsin L structures for comparison. Table 1 Kinetic measurements for intramolecularly quenched fluorogenic (IQF) histone H3 peptide cleavage by cathepsin L. Full size table Table 2 Histone H3 Leu20 recognition by cathepsin L is essential for its cleavage by cathepsin L. Full size table Table 3 Apparent K i values for Z-LR-Mca cleavage by cathepsin L in the presence of the H3 14–31 peptides with various modifications. Full size table The ability of alternative histone-derived peptides to compete with Z-LR-Mca turnover by cathepsin L was also assessed. Peptides derived from a leucine-containing region of the human histone H4 tail are also potential substrates of cathepsin L, though to a much lesser extent than that observed for longer H3-derived peptides ( Supplementary Table S1 ). Histone H3 modifications have modest effects on activity To assess the in vitro effect of PTMs, a systematic analysis of the effect of known histone H3 modifications on cathepsin L activity was undertaken. In assays using either IQF substrates or competitors for Z-LR-Mca, acetylation of H3K18 resulted in a modest reduction in activity for the H3 14−31 peptide ( Tables 1 and 3 , Supplementary Tables S1 and S2 ). Methylation of H3K27 or acetylation of H3Lys14 and H3Lys23 have little impact on either Z-LR-Mca cleavage or the turnover of IQF substrates, though the introduction of an acetyl group at H3Lys18 on peptides carrying other modifications also results in a modest reduction of H3-substrate fitness ( Supplementary Table S1 ). Longer H3 peptides consistently perform as the best competitors for the synthetic substrate ( Supplementary Table S1 ). These trends hold true for assays carried out at either pH 6.0 or 7.4, though the absolute value of the degree of inhibition is reduced at pH 7.4 ( Table 2 ). To date, crystallographic work has centred on inhibitor-bound complexes of mature, active cathepsin L, as well as on the structures of inactive cathepsin mutants with intact prosegments [18] , [19] , [20] , [21] , [22] . In this work, we have generated the mature form of the inactive cathepsin L C25A mutant by means of intermolecular processing of the prosegment by the wild-type protease. We refer to this form of mature protease as mC25A. Subsequent inhibitor treatment and purification completely removed the wild-type activity from the sample and thus enabled, for the first time, cocrystallization with a substrate peptide. As previous research has identified the H3 histone tail as a novel in vivo target of cathepsin L in differentiating murine embryonic stem cells, we have determined the X-ray crystal structures of the apo and H3 19−33 peptide-bound forms of mC25A. The papain-like cysteine proteases, including cathepsin L, possess substrate-binding pockets that can be divided into seven binding subsites, S4 to S3′, that interact with distinct amino acids of the target substrate and confer substrate specificity. Extensive investigations of cathepsin L substrate specificity have identified a strong preference for hydrophobic residues in the S2 subsite, with some preference for positively charged residues in the S1 subsite. Little substrate discrimination is typically observed for the S3 and S4 subsites. The binding of H3 19−33 by mC25A is in agreement both with the S2 subsite preference for hydrophobic residues (H3L20) and with the in vivo and in vitro cleavage data that identified the A21–T22 peptide bond as the primary site of H3 hydrolysis by cathepsin L [16] . The orientation of H3L20 is also consistent with the predicted mode of canonical substrate recognition derived from extensive studies of cathepsin L inhibitor ( Fig. 2 ) [18] , [19] , [21] , [22] , [23] , [24] , [25] . The importance of leucine recognition by the S2 pocket is further highlighted by the loss of competitive inhibition observed for the H3 14−31 L20A and H3 14−31 Q19A/L20A mutant peptides in our assay. Leucine recognition by the S2 subsite may also underlie the substrate turnover observed when cathepsin L is presented with leucine-containing peptides derived from the histone H4 tail. Furthermore, the loss of competitive inhibition on mutation of L20A also suggests that alternative peptides originating from cleavage of other peptide bonds between A21 and S28 of the H3 tails [16] arise from the intrinsic but secondary exopeptidase activity of cathepsin L and not from the primary cleavage of alternative sites. Hence, the initiation of histone H3 cleavage at the A21–T22 bond and subsequent removal of additional residues from the C-terminal peptide of the histone H3 generated the six histone H3 peptide populations that begin with T22, K23, A24, A25, K26 and S28 [16] . Consistently, we have determined the structure of mC25A in complex with the H3 19−33 peptide from several different crystals, but have not captured alternative residues in the S2 subsite, thus supporting A21–T22 peptide bond as the primary and initial site of catalysis. Figure 2: Structural and sequence alignment of inhibitors and substrate sequences in the cathepsin L cleft. ( a ). Superimposition of the H3 19−33 (cyan) peptide with the cathepsin L inhibitors, AZ12878478 (yellow, PDB 3HHA ), and S-benzyl-N-(biphenyl-4-ylacetyl)- L -cysteinyl-N′5′-(diaminomethyl)- D -ornithyl-N-(2-phenylethyl)- L -tyrosinamide (orange, PDB 3BC3 ). In addition to the AZ12878478, an acetate ion aligning with the catalytic residues and a polyethylene moiety in the prime region were also modelled. ( b ) Sequence alignments of selected cathepsin L substrates as identified by mass spectrometry. Each protein target is subject to multiple site of cleavage with both canonical and atypical substrate recognition by the S2 pocket, though consistently there is preference for large and bulky hydrophobic side chains at the S2 site. Full size image Of significant note from a structural perspective is the lack of electron density observed for the substrate residues in the primed region. Although much speculation has pointed to a high-affinity interaction between the substrate and cathepsin L through the primed region, this has neither been experimentally verified nor is necessarily required for efficient substrate recognition by cathepsin L. Of the confirmed biologically relevant substrates for this enzyme, few exhibit significant sequence conservation through the primed region, and systematic analysis of substrate preference by the S1′ subsite has suggested little substrate discrimination [26] . Rather, as supported by the development of cathepsin L inhibitors and their respective optimization for primed region compatibility, the primed sites, including the S1′ region, have shown remarkable little preference for the chemical character of the interacting partner ( Fig. 2b ), and many inhibitor complex structures yield poor electron density in this region ( Fig. 2 ) [18] , [19] , [23] , [25] . The lack of selectivity in primed site recognition is further underscored by the variety of synthetic substrates available for cathepsin L activity assays. Such substrates are typically composed of modified peptides whereby various substituents, including nitroanilides, naphthylamides and amido methylcoumarins, are employed for binding in the primed region. The negligible impact of acetylation of H3K23 on in vitro proteolytic activity, in our work and that of others [14] , is also consistent with a highly accommodating prime region. Despite the remarkable promiscuity observed for the majority of the substrate-binding subsites, enzyme–substrate interactions away from the active-site cleft also may be important in catalysis. In our assays, longer peptides consistently inhibit the turnover of commercial Z-LR-Mca to a greater extent than shorter peptides containing the H3-QLAT primary cleavage site. Extension of the N-terminus of the substrate peptide, exemplified by the H3 14−31 and H3 19−33 peptides reported here, results in the inclusion of a positively charged stretch of amino acids (K 14 APRK 18 ). These H3 residues may interact with a highly negatively charged region proximal to the S3 subsite. The involvement of the S3 subsite and more distant interactions in substrate recognition is also supported by the lower activity of cathepsin L toward leucine-containing peptides from the histone H4 tail. Further structural and biochemical analyses will be essential for determining the relative importance of these more distant interactions in substrate recognition by cathepsin L. With regard to PTMs of the histone tails, the lack of involvement of H3 PTMs in histone cleavage has been suggested previously, as the relative abundance of the peptide populations following cathepsin L cleavage is unchanged in the presence or absence of PTMs along the histone H3 tail [16] . The possibility for modulation of catalytic turnover by acetylation or methylation of H3, however, remains. We have attempted to address this issue by systematically analysing the effect of histone H3 PTMs on the proteolysis of histone H3 peptides as either substrates or competitive inhibitors of synthetic Z-LR-Mca catalysis ( Tables t1 , t2 , t3 ). At both acidic and neutral pH, little effect is observed in either assay employed in this work. Acetylation of H3K23 had no significant effect on the histone H3 peptide proteolysis in our assays, which is in agreement with the aforementioned lack of specific interactions between the primed subsites of cathepsin L and the substrate peptide. Acetylation of H3K18 resulted in only a modest decrease in competitive activity and substrate turnover compared with the unmodified H3 peptide. From a structural perspective, neutralization of the positively charged H3K18 by acetylation weakens its interactions with the negatively charged S3 region. Accordingly, although the S3 subsite can accommodate the negative charges of Asp and Glu residues to some degree, they are less preferred among cathepsin L substrates at this site [27] . This is in contrast to the previous report of the impact of lysine acetylation on H3 cleavage by cathepsin L [16] . Duncan et al . [16] report that acetylation of H3K18 results in a significant increase in peptide cleavage by murine cathepsin L at pH 7.5 when measured using an enzyme-linked immunosorbent assay-based assay with an antibody specific to the primary H3 A21–T22 cleavage product, although this increase is not significant at acidic pH [16] . Our IQF kinetic assays using the murine cathepsin L orthologue, however, showed a similar trend in activity to that of the human cathepsin L ( Table 1 ). In our assays, murine cathepsin L is significantly less active than the human counterpart, but its enzymatic activity is also minimally affected by the introduction of an acetyl group on H3K18 and exhibits no significant response to acetylation at H3K23 or methylation on H3K27. In the human genome, there are two similar proteases that had been called cathepsin L. The original cathepsin L was first isolated in the late 1970s [28] . In 1998, a second human protease was cloned [29] , which was first named as cathepsin L2 but is now referred to as cathepsin V. Human cathepsin V is very similar to cathepsin L in sequence ( Fig. 3 ). The genes for human cathepsin V and cathepsin L are in close proximity on chromosome 9, hinting that they might come from recent gene duplication. In the case of the mouse, it seems that only one cathepsin L form exists, and it is intermediate between human cathepsin V and the original cathepsin L, suggesting that both human genes have diverged since division from the common ancestor of rodent and primate lineages. It has been shown before that human cathepsin V is much less active than human cathepsin L on the usual cathepsin L synthetic substrates [30] . Similar to human cathepsin V, the murine cathepsin L is also much less active than human cathepsin L ( Table 1 ). Although cathepsins L and V have high sequence identities (>70%) and structural similarities ( Fig. 3 ), there are still subtle structural differences along the substrate-binding cleft [31] , which may give rise to the proteolysis activity difference and substrate specificity among these cathepsin enzymes. This warrants further investigation in the future. Figure 3: Sequence and structural conservation among human cathepsins L and V and murine cathepsin L. ( a ) Structure-based sequence alignment of cathepsins L and V. White residues on red background indicate identical residues, red residues on white represent similar residues and the other residues are coloured in black. ( b ) Surface representation of human cathepsins L, V and murine cathepsin L. The structure of murine cathepsin L is modelled based on human cathepsin L. The histone H3 peptide in human cathepsin L complex structure is superimposed to human cathepsin V and murine cathepsin L structures for comparison. Full size image Other factors may be at play in determining the response of cathepsin L to PTMs of the histone H3 tail. Certainly, the possibility of PTM-dependent modulation of cathepsin L activity cannot be excluded and should also be considered within the context of nucleosome and chromatin organization, where PTM will dictate H3 tail accessibility and provide an additional regulatory mechanism for factors associating with the histone tails. The accessibility of cathepsin L cleavage sites, as regulated by histone tail modifications, is consistent with the cell-cycle-dependent proteolysis of the histone tail [14] . Together, the regulatory mechanisms governing tail accessibility and the PTM-dependent modulation of proteolytic cleavage may offer direction over H3 processing by cathepsin L. Protein expression and purification Recombinant human cathepsin L mC25A was produced and purified as previously described [21] , except that 600 nM of active recombinant wild-type cathepsin L (1.7% w active /w inactive ) was used to process the enzyme at 37 °C for 48 h. Wild-type cathepsin L activity was inhibited by the addition of 0.26 mM L - trans -epoxysuccinylleucylamido-(4-guanidino) butane (E-64, Peptide Research Institute). The inactive enzyme was purified by weak cation exchange chromatography. Cathepsin L mC25A free of propeptide eluted at approximately 0.3 M NaCl from a CM Sepharose Fast Flow column using a linear gradient from 0 to 1 M NaCl. Mouse cathepsin L purchased as the pro form from R&D Systems was activated as indicated by the supplier. Activated enzyme was aliquoted and frozen at −70 °C until needed. Peptides All peptides were obtained through the peptide synthesis unit of Tufts University Core Facility. All peptides were verified by mass spectrometry. Fluorescent peptides were synthesized with an amino (N)-terminal fluorescein isothiocyanate (FITC) label, coupled by means of an Ala–His–Ala linker to the desired peptide sequence. IQF peptides were synthesized with N-terminal o -aminobenzoic acid and C-terminal lysine-2,4-dinitrophenylamide conjugates. Crystallization and structure determination Single chain, mature C25A (mC25A) was incubated with a 5 molar excess of each peptide for 30 min at 4 °C. Crystallization conditions were identified by means of sparse matrix screening using the sitting drop vapour diffusion method. The concentration of mC25A was 7 mg ml −1 . Diffraction quality crystals were obtained by mixing equal ratios of protein and reservoir solutions. The final crystallization condition for the apo-mC25A crystals was 0.2 M ammonium sulphate, 0.1 M sodium acetate trihydrate, pH 4.6, 30% polyethylene glycol 2000 monomethylether. Crystals for the mC25A-H3 19−33 complex were obtained in 10% isopropanol, 0.1 M sodium acetate trihydrate, pH 4.0, 22% polyethylene glycol 6000. All crystals were grown at 18 °C and required approximately 4 weeks to reach optimal dimensions. All crystals were soaked in 25% glycerol, added to the final crystallization solution and frozen in liquid nitrogen. Synchrotron diffraction data for the apo-mC25A and mC25A-H3 19−33 crystals were collected at beamline 23-ID-B, Advanced Photon Source, Argonne National Laboratories. All data were indexed and scaled in HKL2000 [32] . Three-dimensional structures were determined by means of molecular replacement with the wild-type cathepsin L structure derived from the PDB 3bc3 deposition using PHASER [33] . Structure building and refinement were carried out with Coot [34] and REFMAC5 [35] , [36] , including TLS (translation, liberation and screw-rotation) refinement with appropriate non-crystallographic restraints. The data collection and structure refinement statistics are presented in Table 4 . Data for the mC25A-H3 19−33 complex were severely anisotropic. Data were collected with 95% completeness in the 2.82–2.69 Å shell and with 78.9% completeness in the 2.69–2.59 Å shell. Owing to the low R merge and high I/sig(I) ratio, data binned in the 2.59–2.5 Å shell were included in the refinement. All structural figures were generated with PyMOL. Table 4 Crystallographic and refinement statistics. Full size table Enzymatic assays Fluorescence measurements were carried out at 25 °C using a Perkin-Elmer LS50B fluorescence spectrophotometer equipped with a thermostatted cuvette holder. The fluorimeter was calibrated before use with a known concentration of Mca. For the substrate benzyloxycarbonyl-leucyl-arginine-Mca (Z-LR-Mca, Novabiochem), the excitation and emission wavelengths were set to 360 and 460 nm, respectively. The slits were set to 10 and 15 nm at the λ ex and λ em , respectively. The concentration of Z-LR-Mca was determined by the fluorescence output upon total hydrolysis with excess protease. The concentration of active wild-type human and mouse cathepsin L was determined by titration with E-64. Before the enzymatic assay, wild-type cathepsin L was activated on ice for 10 min in buffer containing 100 mM Na phosphate pH 6.0 (unless specified) or pH 7.4, 100 mM NaCl, 1 mM EDTA, 0.01% Chaps and 1 mM dithiothreitol. The substrate was prepared in dimethylsulphoxide (DMSO). The FITC-labeled inhibitors were prepared in DMSO whereas the unlabelled peptides were diluted in 100 mM Na phosphate pH 6.0 containing 100 mM NaCl. The overall concentration of DMSO in the cuvette was 3% v/v to ensure substrate and inhibitor solubility. Competitive enzyme assay The overall substrate and inhibitor concentration in the cuvette was 0.16 K m and 25 μM, respectively. The final enzyme concentration was determined to be 48 pM. The reaction was initiated upon addition of enzyme. Initial rates were continuously monitored assuming fast equilibrium. Rates were calculated for <5% substrate conversion for up to 0.5 min. Rates remained constant and linear for at least 11% substrate conversion. Percent inhibition for a given labelled or unlabelled peptide was determined relative to the average rate for the respective two peptides of unrelated sequence. However, the initial rates for the unrelated peptides lacking the FITC label were identical to that with buffer alone. All assays were performed in duplicate. Determination of K i through competitive inhibition The value of the apparent K i (K iapp ) was abstracted from the –X intercept on the linear Dixon plot of 1/v versus [I], where K iapp =−K i × (1+[S]/ K m ). The [S] used was 0.62 μM or 0.16 K m . The concentration of [E] was kept constant at 48.4 pM whereas the [peptide] was varied from 0–66 μM. Initial rates were monitored for <0.5 min, which is <1.4% substrate conversion. All kinetic runs were duplicated and the errors on the reported parameter are <18%. Kinetic measurements with IQF substrates Kinetic measurements on the IQF substrates conjugated at the N-termini with o -aminobenzoic acid and at the C-termini with a lysine-2,4-dinitrophenylamide were carried out as described above, except for the following modifications. The fluorimeter was calibrated with a known concentration of Abz-NH 2 . The increase in fluorescence due to the cleavage of the IQF substrates was measured at λ em 420 nm upon excitation at 320 nm. Inner filter effect was corrected according to Lakowicz et al . [37] ; F corr =F obs × antilog (0.5×(OD ex +OD em )), where F corr and F obs is the corrected and observed fluorescence intensity, and OD ex and OD em is the optical density of the substrate reaction mixture within the cuvette at the excitation and emission wavelengths. The values of k cat and K m were determined by fitting the steady-state rate to a quadratic single binding-site equation in which the change in concentration of both substrate and enzyme upon formation of the enzyme–substrate complex is taken into account [38] . The kinetic parameters were determined using non-linear regression analysis. The calculated k cat / K m values were confirmed for human cathepsin L by fitting a complete progress curve generated under conditions where [S] ≪ < K m to first-order kinetics ( k obs /[E] o = k cat / K m ). [S] was 0.04 K m to at least 9 K m , whereas [E] remained constant at 1.21 nM. Because of the high background fluorescence of the peptides, rates were monitored for <30% total substrate hydrolysis, with an average of 15% conversions. All kinetic runs were duplicated and the errors on the reported parameters are all <25%. With respect to mouse cathepsin L, because of the low error on the fit, [S] ≪ K M can be assumed. Range of [S] used was 21–35 nM with [E]=17.5 nM. Accession codes: Atomic coordinates and structure factors for apo cathepsin L with the C25A mutations and mC25A-H3 19−33 complex have been deposited in the Protein Data Bank under the accession code 3IV2 and 3K24 , respectively. How to cite this article: Adams-Cioaba, M. A. et al . Structural basis for the recognition and cleavage of histone H3 by cathepsin L. Nat. Commun. 2:197 doi: 10.1038/ncomms1204 (2011).